Dynamic histone marks in the hippocampus and cortex facilitate memory consolidation Memory consolidation requires a timely controlled interplay between the hippocampus, a brain region important for memory formation, and the cortex, a region recruited for memory storage. Here we show that memory consolidation is associated with specific epigenetic modifications on histone proteins that have a distinct dynamic in these brain areas. While in the hippocampus, histone post-translational modifications (PTMs) are rapidly and transiently activated after learning, in the cortex they are induced with delay but persist over time. When these histone PTMs are increased in vivo by transgenic intervention or intense training, they facilitate memory consolidation. Conversely, when they are pharmacologically blocked, memory consolidation is impaired. These histone PTMs are further associated with the expression of the immediate early gene zif268 , a transcription factor that favours memory consolidation. These findings reveal the spatiotemporal dynamics of histone marks during memory consolidation, and demonstrate their inherent 'mnemonic' property. Newly formed memory traces need to be stabilized and encoded in neuronal networks to persist for long periods of time. Such stabilization does not occur instantaneously, but depends on memory consolidation, a process that strengthens and maintains initially labile memory traces [1] , [2] . Memory consolidation relies on two major brain regions, the hippocampus and the cortex. While the hippocampus is recruited for the formation and short-term storage of new memory traces, the cortex, in particular the prefrontal cortex (PFC), is needed for long-term storage [3] , [4] , [5] , [6] . At a molecular level, several studies have demonstrated that recent (that is, day-old) memory primarily activates gene expression and metabolic changes in the hippocampus, whereas remote (that is, week-old) memory does so essentially in cortical areas [3] , [7] , [8] . Over the past years, changes in gene expression during memory formation have been shown to be associated with epigenetic processes, in particular post-translational modifications (PTMs) of histone proteins and DNA methylation [9] , [10] , [11] . For histones, several PTMs have been unequivocally linked to memory formation and storage, in particular, phosphorylation of histone (H) 3 serine (S) 10 (refs 12 , 13 , 14 ); acetylation of H2B lysine (K) 5, H3K9, H3K14, H4K5 and H4K12 (refs 10 , 12 , 13 , 14 , 15 , 16 , 17 ); and methylation of H3K36 (ref. 13 ), all of which are marks of transcriptional activation [18] . However, the spatiotemporal dynamics of these histone PTMs in the hippocampus and cortex in relation to memory consolidation remain poorly characterized. Here we show that during object memory consolidation, H3S10 phosphorylation, H3K14 and H4K5 acetylation, and H3K36 trimethylation are rapidly and transiently activated in the hippocampus, while they occur with a delay but persist in the PFC. When these PTMs are increased by transgenic inhibition of protein phosphatase 1 (PP1), a regulator of histone PTMs, or by intense training, memory consolidation is facilitated. In contrast, when their increase is pharmacologically blocked, memory consolidation is prevented. These results identify these histone PTMs as molecular marks necessary for memory consolidation. Hippocampal histone PTMs are induced rapidly but transiently To investigate the association between histone PTMs and memory consolidation, we used an object recognition task in mice. We focused on PTMs previously associated with the formation of long-term associative memory [10] , [12] , [13] , [14] , [15] , [19] , specifically phosphorylation of S10, acetylation of K14 and trimethylation of K36 on histone 3 (H3), and acetylation of K5 on H4. As the formation and storage of object memory depend on a temporally regulated interplay between hippocampal and cortical areas, in particular the PFC [20] , [21] , we postulated that PTMs occur in both brain regions but may be differentially regulated over time. Mice were trained with three unfamiliar objects and tested for their memory for the objects at different intervals after training ( Fig. 1a ). After memory testing (retrieval), the selected PTMs were analysed in the hippocampus in relation to short-term memory (10 min after training, SHORT-TERM), recent memory (1 day after training, RECENT) and remote memory (7 days after training, REMOTE). While all animals had comparable exploration of the three objects during training (Control, Fig. 1b ), they preferentially explored the novel object when tested 10 min later (Control, Fig. 1c ), indicating short-term memory for the familiar objects. At this retention interval, H3S10 phosphorylation (pH3S10), H3K14 acetylation (AcH3K14) and H3K36 trimethylation (3MeH3K36) were significantly increased (by about three- to fourfold) in the hippocampus in trained mice (Control, SHORT-TERM) compared with untrained (but behaviourally habituated, see Methods) animals (Control, HABIT., Fig. 2a–c ). These results suggest a rapid activation of histone PTMs in the hippocampus, consistent with previous reports showing that histone phosphorylation and acetylation are increased shortly after fear conditioning [10] , [12] , [15] . 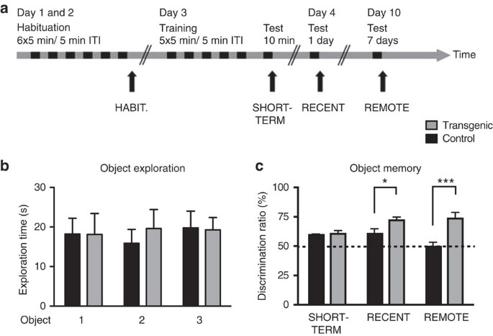Figure 1: Short-term recent and remote object memory in adult mice. (a) Schematic representation of the experimental setup used to elicit object memory in adult mice. Mice were habituated (HABIT.) to an empty arena for six sessions of 5 min with 5 min intertrial intervals (ITI) for 2 days. On day 3, they were trained on five sessions of 5 min with 5 min ITI and tested for short-term memory (SHORT-TERM) after 10 min. For recent memory (RECENT), they were tested after 24 h, and for remote memory (REMOTE), after 7 days. (b) Exploration time in control and transgenic mice for each of the three objects during training shows equal exploration of all objects, indicating no object preference. (c) Black bars, discrimination ratio in control mice 10 min (SHORT-TERM), 1 day (RECENT) and 7 days (REMOTE) after training shows increased exploration of the novel object and significant object memory after 10 min (SHORT-TERM, one-samplet-test,t7=2.50,P<0.05), 1 day (RECENT,t7=2.75,P<0.05), but not after 7 days (REMOTE, not significant). Grey bars, discrimination ratio in transgenic mice show object memory 10 min (SHORT-TERM, one-samplet-test,t7=4.24,P<0.01), 1 day (RECENT,t8=8.45,P<0.001) and 7 days after training (REMOTE,t7=4.98,P<0.01). Asterisks above graphs indicate Bonferronipost-hoctests for multiple comparisons in a two-way analysis of variance with treatment (control or transgenic) and time (SHORT-TERM, RECENT, REMOTE) as the two factors, F2,42=5.51,P<0.01).n=8–9 mice for each time point and group; *P<0.05, ***P<0.001. Error bars are s.e.m. Figure 1: Short-term recent and remote object memory in adult mice. ( a ) Schematic representation of the experimental setup used to elicit object memory in adult mice. Mice were habituated (HABIT.) to an empty arena for six sessions of 5 min with 5 min intertrial intervals (ITI) for 2 days. On day 3, they were trained on five sessions of 5 min with 5 min ITI and tested for short-term memory (SHORT-TERM) after 10 min. For recent memory (RECENT), they were tested after 24 h, and for remote memory (REMOTE), after 7 days. ( b ) Exploration time in control and transgenic mice for each of the three objects during training shows equal exploration of all objects, indicating no object preference. ( c ) Black bars, discrimination ratio in control mice 10 min (SHORT-TERM), 1 day (RECENT) and 7 days (REMOTE) after training shows increased exploration of the novel object and significant object memory after 10 min (SHORT-TERM, one-sample t -test, t 7 =2.50, P <0.05), 1 day (RECENT, t 7 =2.75, P <0.05), but not after 7 days (REMOTE, not significant). Grey bars, discrimination ratio in transgenic mice show object memory 10 min (SHORT-TERM, one-sample t -test, t 7 =4.24, P <0.01), 1 day (RECENT, t 8 =8.45, P <0.001) and 7 days after training (REMOTE, t 7 =4.98, P <0.01). Asterisks above graphs indicate Bonferroni post-hoc tests for multiple comparisons in a two-way analysis of variance with treatment (control or transgenic) and time (SHORT-TERM, RECENT, REMOTE) as the two factors, F 2,42 =5.51, P <0.01). n =8–9 mice for each time point and group; * P <0.05, *** P <0.001. Error bars are s.e.m. 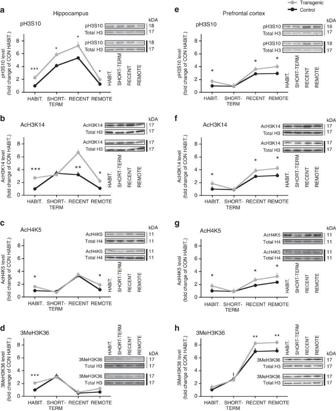Figure 2: Activation of histone PTMs in the hippocampus and PFC. (a–h) Changes in pH3S10, AcH3K14, AcH4K5 and 3MeH3K36 in (a–d) hippocampus and (e–h) PFC in habituated, but untrained (HABIT.) mice, and in mice tested for short-term (SHORT-TERM), recent (RECENT) or remote (REMOTE) memory for both control (black lines) and transgenic animals (grey lines). Representative pictures of western blot analysis are shown adjacent to the line chart. Hippocampus: two-way analysis of variances (ANOVAs), pH3S10, F3, 34=32.31,P<0.001; AcH3K14, F3, 34=21.55,P<0.001; AcH4K5, F3, 34=63.02,P<0.001; 3MeH3K36, F3, 34=58.26,P<0.001. PFC: two-way ANOVAs, pH3S10, F3, 18=12.63,P<0.01; AcH3K14, F3, 18=11.88,P<0.01; AcH4K5, F3, 18=29.44,P<0.001; 3MeH3K36, F3, 18=59.83,P<0.001. Histone PTMs are expressed as fold change to HABIT. animals. Asterisks indicate Bonferronipost-hoctests for the effect of treatment (control or transgenic) at individual time points following two-way ANOVAs with treatment (control and transgenic) and time (HABIT., SHORT-TERM, RECENT and REMOTE) as factors; *P<0.05, **P<0.01, ***P<0.001. Number of animals used for hippocampal samples: control (CON), HABIT.,n=13; SHORT-TERM,n=9; RECENT,n=8; REMOTE,n=8; transgenic, HABIT.,n=10; SHORT-TERM,n=8; RECENT,n=8; REMOTE,n=8; for PFC samples: CON, HABIT.,n=5; SHORT-TERM,n=5; RECENT,n=6; REMOTE,n=6; transgenic, HABIT.,n=6 for SHORT-TERM, RECENT and REMOTE. Error bars are s.e.m. Full size image Figure 2: Activation of histone PTMs in the hippocampus and PFC. ( a – h ) Changes in pH3S10, AcH3K14, AcH4K5 and 3MeH3K36 in ( a – d ) hippocampus and ( e – h ) PFC in habituated, but untrained (HABIT.) mice, and in mice tested for short-term (SHORT-TERM), recent (RECENT) or remote (REMOTE) memory for both control (black lines) and transgenic animals (grey lines). Representative pictures of western blot analysis are shown adjacent to the line chart. Hippocampus: two-way analysis of variances (ANOVAs), pH3S10, F 3, 34 =32.31, P <0.001; AcH3K14, F 3, 34 =21.55, P <0.001; AcH4K5, F 3, 34 =63.02, P <0.001; 3MeH3K36, F 3, 34 =58.26, P <0.001. PFC: two-way ANOVAs, pH3S10, F 3, 18 =12.63, P <0.01; AcH3K14, F 3, 18 =11.88, P <0.01; AcH4K5, F 3, 18 =29.44, P <0.001; 3MeH3K36, F 3, 18 =59.83, P <0.001. Histone PTMs are expressed as fold change to HABIT. animals. Asterisks indicate Bonferroni post-hoc tests for the effect of treatment (control or transgenic) at individual time points following two-way ANOVAs with treatment (control and transgenic) and time (HABIT., SHORT-TERM, RECENT and REMOTE) as factors; * P <0.05, ** P <0.01, *** P <0.001. Number of animals used for hippocampal samples: control (CON), HABIT., n =13; SHORT-TERM, n =9; RECENT, n =8; REMOTE, n =8; transgenic, HABIT., n =10; SHORT-TERM, n =8; RECENT, n =8; REMOTE, n =8; for PFC samples: CON, HABIT., n =5; SHORT-TERM, n =5; RECENT, n =6; REMOTE, n =6; transgenic, HABIT., n =6 for SHORT-TERM, RECENT and REMOTE. Error bars are s.e.m. Full size image When tested for recent memory 1 day after training, the animals still remembered the familiar objects (Control, Fig. 1c ), and at this interval, pH3S10 was further increased in the hippocampus, suggesting a day-long activation of this PTM in relation to memory consolidation. AcH3K14 also remained elevated but did not further increase, whereas AcH4K5 increased at this time point unlike after 10 min. In contrast, 3MeH3K36 decreased and was back to baseline (Control, RECENT, Fig. 2a–d ). For remote memory 7 days after training, however, all hippocampal PTMs decreased back to baseline (Control, REMOTE, Fig. 2a–e ), and memory performance was at chance level ( Fig. 2c ). These results suggest that histone PTMs are rapidly and transiently activated in the hippocampus by learning. While pH3S10 and AcH3K14 are associated with short-term and recent memory, 3MeH3K36 is primarily associated with short-term and AcH4K5 with recent memory. Importantly, the transience of these PTMs is consistent with the postulated time-limited engagement of the hippocampus in the processing of newly formed memory traces [1] , [2] , [7] . Further, the activation of PTMs is selectively associated with memory recall, as none of the PTMs was changed without memory testing ( Supplementary Fig. S1a–e ). Cortical histone PTMs are activated with delay but persist We next examined the dynamics of histone PTMs in the PFC at the same retention intervals. Although the role of the PFC in long-term associative memory is well established [5] , its role in object memory is more putative [21] . Thus, we first tested whether the consolidation of long-term object memory depends on the PFC. We lesioned the medial PFC using ibotenic acid (IA) ( Supplementary Fig. S2a ) before training, and then compared memory performance in lesioned mice with sham-lesioned littermates. Recent memory was not affected by the lesion ( Supplementary Fig. S2b ), but remote memory was impaired in IA-treated animals ( Supplementary Fig. S2c ), suggesting that the medial PFC is needed for remote object memory. We then examined the different histone PTMs in the PFC during memory consolidation. For short-term memory, no significant change in any of the PTMs was detected, although there was a trend for an increase in 3MeH3K36 at this interval (Control, SHORT-TERM, Fig. 2e–h ). In contrast, 1 day after training, all PTMs were significantly increased (Control, RECENT, Fig. 2e–h ), most notably 3MeH3K36, which was about sevenfold higher than in untrained animals (Control, RECENT, Fig. 2h ). Remarkably, for remote memory, all histone PTMs examined were still increased at a level comparable to that 1 day after training (Control, REMOTE, Fig. 2e–h ). These results indicate that the same histone PTMs induced in the hippocampus for short-term and recent memory are established in the cortex, but only after a delay, that is, only for recent and remote memory, and not for short-term memory. This suggests that PTMs in the PFC are more stable than in the hippocampus, and highlights a correlation between the spatiotemporal dynamics of their activation and memory consolidation [3] , [7] , [8] . Enhanced histone PTMs facilitate memory consolidation To further examine the relevance of histones marks for memory consolidation, we took advantage of a recently developed transgenic mouse model [22] , in which memory is enhanced by inhibition of the chromatin regulator and memory suppressor PP1 [23] . In this model, PP1 is selectively inhibited in forebrain neurons, in particular in the hippocampus and PFC ( Supplementary Fig. S3 ) [13] , [14] , [22] . When tested on the object recognition task, the transgenic mice (Transgenic) had memory performance comparable to control mice (Control) 10 min after training but had improved memory both 1 and 7 days after training ( Fig. 1c ), suggesting a positive effect of PP1 inhibition on recent and remote memory, and on memory consolidation. Object exploration during training was comparable for all objects ( Fig. 1b ). These results indicate that facilitated memory consolidation in these mice is accompanied by increased histone PTMs. The analyses of PTMs in untrained, but habituated transgenic mice revealed that pH3S10, AcH3K14 and AcH4K5 are increased in both the hippocampus and PFC, and 3MeH3K36 is increased in the hippocampus (HABIT., grey line, Fig. 2 ). Further, 10 min after training, hippocampal pH3S10 was increased by about threefold compared with untrained animals (SHORT-TERM, grey line, Fig. 2a ), whereas histone acetylation and methylation were not changed in the hippocampus (compared with control mice). However, after 1 day, both pH3S10 and AcH3K14 were increased, and were significantly higher than in controls at the same retention interval (RECENT, grey line, Fig. 2a,b ). AcH4K5 and 3MeH3K36 were increased and decreased, respectively, when compared with untrained transgenic animals, but their level was comparable to controls at the same time point (RECENT, grey line, Fig. 2c,d ). When tested 7 days after training, all PTMs in the hippocampus in the transgenic mice were back to the level in untrained animals (REMOTE, grey line, Fig. 2a–d ). These results indicate that a concomitant increase in pH3S10 and AcH3K14 in the hippocampus is associated with object memory formation in the transgenic mice, consistent with the reported role of these PTMs in fear memory [10] , [12] , [15] . Importantly, the data further suggest a dissociation between histone PTMs in the hippocampus and remote memory, because remote memory was improved after 7 days in the transgenic animals despite no apparent change in hippocampal PTMs compared with untrained mice. This raises the possibility that cortical PTMs are involved. To investigate this possibility, we examined PTMs in the PFC in the transgenic mice. Although none of the PTMs was changed after 10 min, they were all significantly increased after 1 day (SHORT-TERM and RECENT, grey line, Fig. 2e–h ), and this increase persisted for 7 days (REMOTE, grey line, Fig. 2e–h ). Importantly, histone PTMs in PFC in the transgenic mice were significantly higher 1 and 7 days after training than in controls, and this correlated with a selective improvement in recent and remote memory in the transgenic mice ( Fig. 1c ). Together, these results confirm that histone marks in the cortex have a delayed onset, and suggest that the parallel activation of pH3S10, AcH3K14, AcH4K5 and 3MeH3K36, and their occurrence first in the hippocampus, then in the PFC not only accompany but also promote the consolidation of long-term memory. To confirm this hypothesis in physiologically relevant conditions, we used an intensive training protocol (15 min instead of 5 min intertrial intervals) known to elicit robust long-term memory [23] , and trained a new batch of control mice ( Fig. 3a ). Memory was tested 7 days later. This training resulted in significantly enhanced histone PTMs on pH3S10, AcH3K14 and 3MeH3K36 in the PFC, with the exception of AcH4K5 ( Fig. 3b–f ), and, importantly, in a robust improvement of remote memory performance ( Fig. 3g ). Taken together, these findings suggest that the degree of pH3S10, AcH3K14 and 3MeH3K36 might determine how well a memory trace is consolidated. 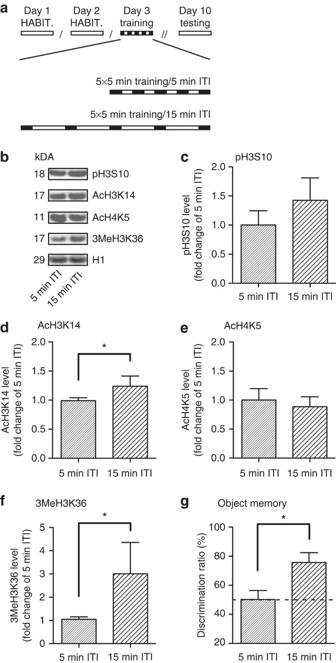Figure 3: Intense training enhances histone PTMs and memory consolidation. (a) Scheme of the different training protocols used to elicit weak or strong object memory in control mice. ITI, intertraining interval. (b) Representative pictures of western blot analyses of histone PTMs 7 days after training in the 15 min-ITI group compared with the 5 min-ITI group. (c) pH3S10, not significant (n.s.); (d) AcH3K14,t12=1.73,P≤ 0.05; (e) AcH4K5, n.s.; (f) 3MeH3K36,t11=2.27,P≤ 0.05. (g) Discrimination ratio 7 days after training showing enhanced REMOTE memory in the 15 min-ITI group compared with the 5 min-ITI group (n=11–16 animals per group), Student'st-test,t24=1.9,P≤ 0.05.Error bars are s.e.m. Figure 3: Intense training enhances histone PTMs and memory consolidation. ( a ) Scheme of the different training protocols used to elicit weak or strong object memory in control mice. ITI, intertraining interval. ( b ) Representative pictures of western blot analyses of histone PTMs 7 days after training in the 15 min-ITI group compared with the 5 min-ITI group. ( c ) pH3S10, not significant (n.s. ); ( d ) AcH3K14, t 12 =1.73, P ≤ 0.05; ( e ) AcH4K5, n.s. ; ( f ) 3MeH3K36, t 11 =2.27, P ≤ 0.05. ( g ) Discrimination ratio 7 days after training showing enhanced REMOTE memory in the 15 min-ITI group compared with the 5 min-ITI group ( n =11–16 animals per group), Student's t -test, t 24 =1.9, P ≤ 0.05.Error bars are s.e.m. Full size image The inhibition of histone PTMs impairs object memory To examine whether the observed histone PTMs are causally linked to object memory formation, we blocked their activation in vivo using a cocktail of inhibitors containing staurosporine, a blocker of H3-specific kinases [24] , C646, an inhibitor of the histone acetyltransferase p300/CBP [25] , and 3-deazaneplanocin A, an inhibitor of histone methyltransferases [26] . These inhibitors effectively blocked histone phosphorylation, acetylation and methylation in the brain ( Fig. 4a–d ). Crucially, when animals treated with these inhibitors were tested, remote object memory was impaired ( Fig. 4e ). These findings show that without an increase in histone phosphorylation, acetylation and methylation, object memory cannot efficiently consolidate, and thus provide a causal link between histone PTMs and memory consolidation. 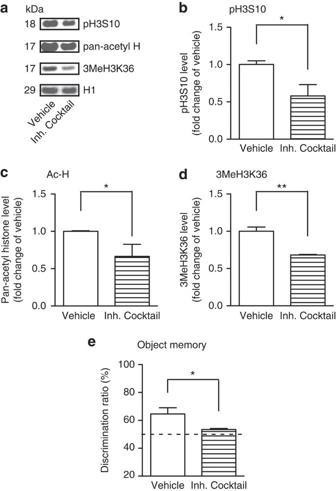Figure 4: Blocking the activation of histone PTMs prevents memory retention. (a) Discrimination ratio in animals injected with the histone PTM inhibitor (Inh) cocktail (n=4) or vehicle (vehicle,n=8) 7 days after training on the object-recognition task. Remote memory is impaired when histone PTMs are blocked. Student'st-test,t10=1.75,P≤ 0.05. (b) Representative western blot images of histone PTMs 1 day after training in animals injected with the inhibitor cocktail (n=4) show reduced histone PTMs compared with vehicle-injected animals (n=8). (c) Quantification of pH3S10,t6=2.63,P≤ 0.05; (d) Quantification of pan-acetyl histone,t7=1.82,P≤ 0.05; (e) Quantification of 3MeH3K36,t5=4.67,P≤ 0.01. Error bars are s.e.m. Figure 4: Blocking the activation of histone PTMs prevents memory retention. ( a ) Discrimination ratio in animals injected with the histone PTM inhibitor (Inh) cocktail ( n =4) or vehicle (vehicle, n =8) 7 days after training on the object-recognition task. Remote memory is impaired when histone PTMs are blocked. Student's t -test, t 10 =1.75, P ≤ 0.05. ( b ) Representative western blot images of histone PTMs 1 day after training in animals injected with the inhibitor cocktail ( n =4) show reduced histone PTMs compared with vehicle-injected animals ( n =8). ( c ) Quantification of pH3S10, t 6 =2.63, P ≤ 0.05; ( d ) Quantification of pan-acetyl histone, t 7 =1.82, P ≤ 0.05; ( e ) Quantification of 3MeH3K36, t 5 =4.67, P ≤ 0.01. Error bars are s.e.m. Full size image PTMs are increased at the zif268 gene during consolidation Immediate early genes such as zif268 are known to be activated during memory consolidation for both object [27] , [28] and fear memory [3] , [8] . We therefore examined whether the changes in histone PTMs are associated with altered zif268 expression in relation to object memory consolidation. We first measured the level of zif268 mRNA in the hippocampus and PFC in control mice 1 (RECENT) and 7 days (REMOTE) after training. Z if268 expression was increased in the hippocampus but not in the PFC after 1 day. However, after 7 days, it was back to baseline in the hippocampus but increased in the PFC ( Fig. 5a,f , black line), suggesting a selective upregulation of zif268 expression in the hippocampus for recent memory and in the PFC for remote memory. Consistent with the lack of change in histone PTMs without retrieval, the level of zif268 mRNA was not altered 1 day after training alone ( Supplementary Fig. S1f ). This corroborates previous findings showing selective upregulation of zif268 mRNA during retrieval [29] . 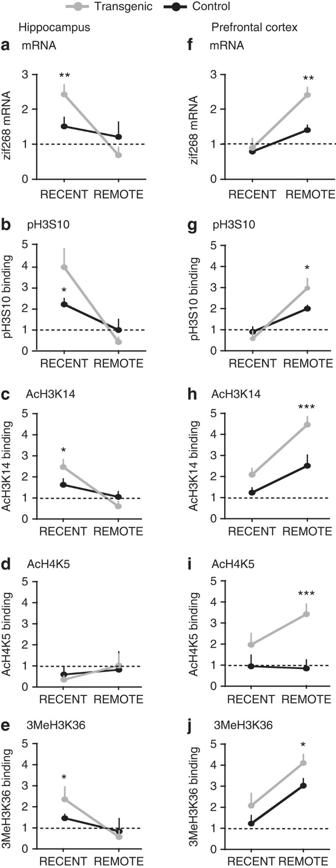Figure 5: Memory consolidation is associated withzif268expression and increased histone PTMs. zif268mRNA expression and promoter occupancy in the hippocampus (a–e) and PFC (f–j) 1 day (RECENT) and 7 days (REMOTE) after training on the object-recognition task in control (black,n=3) and transgenic mice (grey,n=3).zif268mRNA expression in (a) hippocampus: inter-group comparison at each retention interval; RECENT, transgenic versus control, Student'st-test,t4=4.384,P<0.01; REMOTE, not significant (n.s.); and (f) PFC: inter-group comparison at retention interval; RECENT, n.s., REMOTE, transgenic versus control,t4=5.671,P<0.01;zif268promoter occupancy by pH3S10 in (b) hippocampus: inter-group comparison at each retention interval; RECENT, transgenic versus control,t4=3.393,P<0.05; REMOTE, n.s.; and (g) PFC: inter-group comparison at each retention interval; RECENT, n.s., REMOTE, transgenic versus control,t4=2.163,P<0.05; by AcH3K14 in (c) hippocampus: inter-group comparison at each retention interval; RECENT, transgenic versus control,t4=2.091,P<0.05; REMOTE, n.s.; and in (h) PFC: inter-group comparison at each retention interval; RECENT, transgenic versus control,t4=3.82,P<0.01, REMOTE, transgenic versus control,t4=4.818,P<0.01; by AcH4K5 in (d) hippocampus, all n.s.; and in (i) PFC: inter-group comparison at each retention interval; RECENT, n.s., REMOTE, transgenic versus control,t4=8.419,P<0.001; by 3MeH3K36 in (e) hippocampus: intergroup comparison at each retention interval; RECENT, transgenic versus control,t4=2.388,P<0.05; REMOTE, n.s.; and in (j) PFC: Inter-group comparison at each retention interval; RECENT, n.s., REMOTE, transgenic versus control,t4=3.235,P<0.05; All values are expressed as fold change of habituated control animals. Error bars are s.e.m. Figure 5: Memory consolidation is associated with zif268 expression and increased histone PTMs. zif268 mRNA expression and promoter occupancy in the hippocampus ( a – e ) and PFC ( f – j ) 1 day (RECENT) and 7 days (REMOTE) after training on the object-recognition task in control (black, n =3) and transgenic mice (grey, n =3). zif268 mRNA expression in ( a ) hippocampus: inter-group comparison at each retention interval; RECENT, transgenic versus control, Student's t -test, t 4 =4.384, P <0.01; REMOTE, not significant (n.s. ); and ( f ) PFC: inter-group comparison at retention interval; RECENT, n.s., REMOTE, transgenic versus control, t 4 =5.671, P <0.01; zif268 promoter occupancy by pH3S10 in ( b ) hippocampus: inter-group comparison at each retention interval; RECENT, transgenic versus control, t 4 =3.393, P <0.05; REMOTE, n.s. ; and ( g ) PFC: inter-group comparison at each retention interval; RECENT, n.s., REMOTE, transgenic versus control, t 4 =2.163, P <0.05; by AcH3K14 in ( c ) hippocampus: inter-group comparison at each retention interval; RECENT, transgenic versus control, t 4 =2.091, P <0.05; REMOTE, n.s. ; and in ( h ) PFC: inter-group comparison at each retention interval; RECENT, transgenic versus control, t 4 =3.82, P <0.01, REMOTE, transgenic versus control, t 4 =4.818, P <0.01; by AcH4K5 in ( d ) hippocampus, all n.s. ; and in ( i ) PFC: inter-group comparison at each retention interval; RECENT, n.s., REMOTE, transgenic versus control, t 4 =8.419, P <0.001; by 3MeH3K36 in ( e ) hippocampus: intergroup comparison at each retention interval; RECENT, transgenic versus control, t 4 =2.388, P <0.05; REMOTE, n.s. ; and in ( j ) PFC: Inter-group comparison at each retention interval; RECENT, n.s., REMOTE, transgenic versus control, t 4 =3.235, P <0.05; All values are expressed as fold change of habituated control animals. Error bars are s.e.m. Full size image Next, we examined the relationship between zif268 expression and PTMs associated with memory consolidation. pH3S10, AcH3K14, AcH4K5 and 3MeH3K36 were measured at the promoter region of zif268 by chromatin immunoprecipiation (ChIP). In control mice 1 day after training, pH3S10, AcH3K14 and 3MeH3K36 were significantly increased at the zif268 promoter in the hippocampus ( Fig. 5b,c,e , RECENT, black line), but not in the PFC ( Fig. 5g,h,j , RECENT, black line). However, after 7 days, pH3S10, AcH3K14, and 3MeH3K36 were back to baseline in the hippocampus ( Fig. 5b,c,e , REMOTE, black line), but still significantly increased in the PFC ( Fig. 5g,h,j , REMOTE, black line). AcH4K5, however, did not change ( Fig. 5d,i , black line), suggesting that this mark is not involved in zif268 regulation. Together, these findings suggest a combined activation of pH3S10, AcH3K14 and 3MeH3K36 at the zif268 promoter in relation to zif268 expression during memory consolidation. Enhanced zif268 histone PTMs and facilitated consolidation Finally, we examined whether zif268 mRNA expression and promoter-associated histone PTMs are associated with facilitated memory consolidation in the transgenic mice. Consistent with the enhanced recent and remote memory, zif268 expression was significantly higher in the hippocampus of transgenic animals compared with controls 1 day but not 7 days after training ( Fig. 5a , grey line). In the PFC, however, it was higher than in control mice 7 days after training ( Fig. 5f , grey line). These findings support the hypothesis that the extent of zif268 expression in the hippocampus and cortex correlates with memory performance. Further, ChIP analyses revealed that pH3S10, AcH3K14 and 3MeH3K36 are significantly enriched at the zif268 promoter in the hippocampus in transgenic mice 1 day after training ( Fig. 5b,c,e , RECENT, grey line), consistent with the increased zif268 expression at this time point ( Fig. 5a , RECENT, grey line). In contrast in the PFC, pH3S10, AcH3K14 and 3MeH3K36 were not changed 1 day after training ( Fig. 5g,h,j , RECENT, grey line), in line with unchanged zif268 expression ( Fig. 5f , RECENT, grey line). Notably, 7 days after training, no increase in pH3S10, AcH3K14 or 3MeH3K36 was observed in the hippocampus ( Fig. 5b,c,e , REMOTE, grey line), whereas in the PFC, pH3S10, AcH3K14 and 3MeH3K36 were significantly enriched at zif268 promoter ( Fig. 5g,h,j , REMOTE, grey line). As in control mice, AcH4K5 remained unchanged after 1 day, but was increased in PFC after 7 days ( Fig. 5d,i , grey line), suggesting that this residue is likely not critical for zif268 expression. Taken together, these data indicate that recent and remote object memory is associated with dynamic changes in pH3S10, AcH3K14 and 3MeH3K36 at the zif268 promoter, which parallels zif268 expression during memory consolidation. Moreover, the data show that increased histone PTMs at zif268 promoter, an immediate early-gene important for memory formation and storage [30] , correlate with facilitated memory consolidation. The present findings show the spatiotemporal dynamics of specific histone PTMs in the hippocampus and PFC during memory consolidation. Histone PTMs are first established in the hippocampus where they are transient, and are later induced in the cortex, where they persist for up to 7 days. The data identify H3S10 phosphorylation and H3K14/H4K5 acetylation in the hippocampus as being associated with recent memory, and H3S10 phosphorylation, H3K14/H4K5 acetylation and H3K36 trimethylation in the PFC associated with remote memory consolidation. Mimicking these PTMs in forebrain neurons in adult mice by transgenic intervention or intensive training favours memory retention, whereas blocking these PTMs abolishes memory. These findings strongly suggest that PTMs act as 'mnemonic' epigenetic marks that accompany the consolidation of memory traces from hippocampal to cortical areas. The data also show that these marks occur at the zif268 promoter and correlate with a shift of zif268 expression from the hippocampus to the PFC as the memory matures, suggesting an important functional role of these histone PTMs in memory consolidation. The results are in line with several recent findings showing that enhancing histone acetylation favours memory, including object [13] , [31] , fear [10] , [12] , [14] , [15] , [17] , [32] , [33] , [34] , spatial [13] , [34] and taste [19] , [35] memory. They significantly extend these findings by showing that in addition to histone acetylation, histone phosphorylation and methylation (on H3K36) are activated in a temporally and spatially regulated manner during memory consolidation in both the hippocampus and the cortex. Importantly, they provide the first evidence of a simultaneous activation of these marks and the necessity of their combined activation for the successful consolidation of a memory trace. Remarkably, the time course of the establishment of these histone PTMs in the hippocampus and the cortex recapitulates the dynamics of memory consolidation. For short-term memory, which is hippocampus-dependent, histone PTMs peak solely in the hippocampus. In contrast, for recent memory, which still engages the hippocampus but progressively recruits cortical areas as well [36] , histone PTMs are increased in both brain areas, whereas for hippocampus-independent remote memory, histone PTMs are activated only in the PFC. These epigenetic modifications may therefore be conceived as molecular mnemonics, a concept fostered by the findings that upon intense training, these marks are enhanced together with memory consolidation. This is also in line with the proposal by Lesburguères et al . [19] that upon first encounter with a novel stimulus, a subset of neurons in the hippocampus and olfactory cortex are 'tagged' by histone acetylation, which favours memory consolidation and the interplay between the hippocampus and the cortex during this period. In perspective, as histones can carry many PTMs in the brain [37] , [38] , [39] , additional PTMs such as sumoylation or ubiquitination may constitute additional molecular mnemonics. Memory consolidation may also be supported by the combined action of histone PTMs and DNA methylation, another epigenetic modification shown to be involved in memory formation [11] . Exploring these possibilities and potential ways to favour such mnemonic marks by natural or pharmacological cognitive strategies should be of great interest for future studies. Animals Adult (3–6 months old) male double transgenic mice carrying a fragment including amino acids 143 to 224 of the nuclear inhibitor of PP1 (NIPP1*) linked to a bidirectional tetO (BiTetO) promoter with a LacZ reporter gene (Transgenic) were used as described [22] . To obtain double transgenic animals, these mice were crossed with mice expressing a reverse tetracycline-controlled transactivator (rtTA2) under the control of the forebrain-specific CaMKIIα promoter [40] . Control mice were carrying no transgene or either one of the transgenes. All mice were fed dox. For experiments involving experimental manipulations (see below), C57Bl/6 adult wild-type males were used. All animals were maintained in accordance with the Federation of Swiss Cantonal Veterinary Office and INSERM committee or European Community Council Directive (86/609/EEC) guidelines, or the Massachusetts Institute of Technology's Division of Comparative Medicine guidelines. Behaviour The novel object-recognition task was conducted essentially as described [13] . Training consisted in exposing the animals five times for 5 min to the objects, with either a 5 min or a 15 min intertrial interval (see Figs 1a and 3a ). Time spent with the objects was measured using an automated animal tracking system (Viewpoint). A discrimination ratio (DR) was calculated as DR= t novel /( t novel +( t familiar1 + t familiar2 )/2), where t novel is the time spent with the novel object (seconds) and t familiar is the time spent with familiar objects 1 and 2 (seconds). As baseline for all molecular analyses, '' mice, which are animals that went through a 2-day habituation phase, but never exposed to any object and not trained, were used. Short-term memory (SHORT-TERM) was assessed 10 min after training. For recent memory (RECENT), mice were tested 24 h after training. For remote memory (REMOTE), mice were tested 7 days after training. Note that animals were only tested for one time point after training, then they were killed (see below). Experimental manipulations To simultaneously block histone PTMs, wild-type mice were injected i.p. with a phosphatase/histone acetyl transferase/histone methyl transferase inhibitor cocktail consisting of 0.2 mg kg −1 staurosporine (Cell Signaling), a kinase inhibitor that co-targets H3 kinases [24] , 10 nmol C646 (Tocris Bioscience), an inhibitor of the histone acetyl transferase p300/CBP [25] , and 2 mg kg −1 3-deazaneplanocin A (Cayman), an inhibitor of histone methyltransferases [26] . The drugs were prepared in dimethylsulphoxide (Sigma). Control, that is, non-treated animals received the same volume of dimethylsulphoxide (in 0.9% saline). The animals received single doses of the drugs cocktail daily on four consecutive days, starting immediately after object-recognition training. Remote object memory was assessed 7 days later. For lesion experiments on PFC, wild-type mice under deep anaesthesia (100 mg kg −1 ketamine/10 mg kg −1 xylazine) were stereotaxically injected with 0.5 μl of IA (Sigma) at a rate of 0.1 μl min −1 bilaterally into the medial PFC (anterior–posterior 1.98 mm, medial–lateral 0.25 mm from bregma, dorsoventral −1.08 mm from the dura). Needles were left in place for an additional 5 min to assure even distribution. Mice were allowed to recover for 14 days before behavioural testing. Samples preparation For western blotting, RT–PCR and ChIP, animals were sacrificed by cervical dislocation after behavioural testing, their brain was dissected, snap-frozen and stored at −80 °C until further processing. For hippocampal samples, the entire hippocampus was used. For PFC samples, the medial part of PFC (anterior 2.8 mm to posterior 1.78 mm, medial–lateral ±0.6 mm, dorsoventral −2.0 mm from dura) was used. Animals for immunohistochemistry were transcardially perfused with 10% paraformaldehyde (Electron Microscopy Sciences) under deep anaesthesia (100 mg kg −1 ketamine/10 mg kg −1 xylazine), and their brain was coronally sectioned at 40 μm thickness using a vibratome (Leica). Western blotting Western blotting was performed as previously described [13] . Briefly, 10–15 μg proteins from nuclear extracts were resolved on 10–12% SDS–PAGE and transferred onto a nitrocellulose membrane (Bio-Rad). Membranes were blocked (Rockland IR blocking buffer, Rockland) then incubated in primary and secondary antibodies. Band intensity was determined and quantified using an Odyssey IR scanner (Li-Cor Biosciences). Values at different retention interval after training, and values in transgenic mice were normalized to values in control littermates before training. The following antibodies were used: H3 (1:2,000), H4 (1:2,000; Millipore); phospho H3S10 (1:1,000), pan-acetyl H3 (1:1,000) acetyl H3K14 (1:1,000), acetyl H4K5 (1:1,000; Millipore); trimethyl H3K36 (1:1,000), H1.0 (1:1,000; Abcam); goat anti-rabbit (IRDye 680 nm, 1:10,000) and goat anti-mouse (IRDye 800 nm, 1:10,000; Li-Cor Biosciences). Samples from different conditions were processed on the same blots whenever possible. For samples processed on different blots, a standard weight loading control (Bio-Rad) was used on each blot, and band intensity was used for normalization to ensure accuracy between blots. Histone H1.0 was used as an internal control. All histones PTMs are expressed as fold change to untrained, but habituated control animals and normalized to total core histone level (either H3 or H4) or to histone H1.0. RT–PCR RT–PCR was performed as described previously [13] . Total RNA was extracted using the NucleoSpin Kit II (Macherey-Nagel), purified with RQ1 DNase (Promega), and reverse-transcribed using the SuperScript First-Strand Synthesis System for RT–PCR II (Invitrogen). For the assessment of the transgene expression, the following primers were used: NIPP1: forward, 5′-TGACATCCACTTTGCCTTTCTCTC-3′; reverse, 5′- CAACCCAGAGGATGTGGATC-3′; LacZ: forward, 5′-TTCACTGGCCGTCGTTTTACAACGTCGTGA-3′; reverse, 5′-ATGTGAGCGAGTAACAACCCGTCGGATTCT-3′; GAPDH: forward, 5′-ACCACAGTCCATGCCATCA-3′; reverse, 5′-CACCACCCTGTTGCTGTAGCC-3′. For the assessment of zif268 mRNA level, gene-specific Taqman probes were used for zif268 and GAPDH (Applied Biosystems). Values were normalized to GAPDH and the quantitative Ct-method was used for quantification of relative expression level [41] . Chromatin immunoprecipitation ChIP was performed as described previously [13] with the same antibodies as above. In brief, after crosslinking with formaldehyde (Sigma), samples were collected and washed twice in ice-cold PBS containing proteinase inhibitors (Complete, Roche), homogenized in cell lysis buffer containing proteinase and phosphatase inhibitors (1 mM β-glycerophosphate, 10 mM NaF, 0.1 mM Na 3 VO 4 ), then in nuclear lysis buffer containing the same proteinase and phosphatase inhibitors. Samples were sonicated on ice using a Branson Digital Sonifier with 15 cycles at 50% power setting of 10 s each. A total of 100 μg per sample were used for each ChIP reaction in IP buffer (0.1% SDS, 1% Triton X-100, 150 mM NaCl, 2 mM EDTA pH 8, 20 mM Tris–Cl pH 8.0 containing the same inhibitors) and immunoprecipitated overnight at 4 °C with 5 μg of antibodies. After IP, DNA–histone complexes were collected in 40 μl of 10% BSA/salmon sperm DNA (Stratagene)-precleared Protein A/Sepharose Beads (GE Healthcare) for 2 h at 4 °C. The sample/bead mixtures were washed twice with wash buffer (0.1% SDS in IP buffer), once with final wash buffer (0.1% SDS, 1% Triton X-100, 0.5 M NaCl, 2 mM EDTA pH 8.0, 20 mM Tris–Cl pH 8.0 containing proteinase inhibitors), and twice with TE (10 mM Tris–Cl pH 8.0, 1 mM EDTA). DNA and histones were dissociated by incubation in 1% SDS in TE for at least 4 h at 65 °C. Finally, proteins were digested with proteinase K (Sigma) for 1 h at 45 °C and the DNA extracted with phenol/chloroform/isoamyl alcohol (Fluka) and resuspended in 100 μl TE. ChIP experiments were run at least in biological triplicates. Immunoprecipitated DNA was amplified on a thermal cycler (Applied Biosystems) using SYBR green (Bio-Rad) and the following primers for zif268: forward, 5′-GTGCCCACCACTCTTGGAT-3′; reverse, 5′-CGAATCGGCCTCTATTTCAA-3′. Values were normalized to total DNA input. Immunohistochemistry Slices were permeabilized with 0.1% Triton X-100 in PBS, blocked and incubated with 0.1% Triton-X100/10% fetal bovine serum in PBS with NeuN (1:1,000, Chemicon), and visualized with a Cy3 secondary antibody (1:400, Molecular Probes), and Hoechst 33342 (1:1,000, Invitrogen) on a Zeiss LSM510 confocal microscope. Statistics Two-way analysis of variances followed by Bonferroni post-hoc comparisons or two-sample t -tests were used to determine time and treatment effect. One-sample t -tests were conducted to compare means per group to a hypothetical value. Statistical significance was set at * P ≤ 0.05, ** P ≤ 0.01 and *** P ≤ 0.001. All values are expressed as mean±s.e.m. How to cite this article: Gräff, J. et al . Dynamic histone marks in the hippocampus and cortex facilitate memory consolidation. Nat. Commun. 3:991 doi: 10.1038/ncomms1997 (2012).